The oncogenic transcription factor c-Jun regulates glutaminase expression and sensitizes cells to glutaminase-targeted therapy Many transformed cells exhibit altered glucose metabolism and increased utilization of glutamine for anabolic and bioenergetic processes. These metabolic adaptations, which accompany tumorigenesis, are driven by oncogenic signals. Here we report that the transcription factor c-Jun, product of the proto-oncogene JUN , is a key regulator of mitochondrial glutaminase (GLS) levels. Activation of c-Jun downstream of oncogenic Rho GTPase signalling leads to elevated GLS gene expression and glutaminase activity. In human breast cancer cells, GLS protein levels and sensitivity to GLS inhibition correlate strongly with c-Jun levels. We show that c-Jun directly binds to the GLS promoter region, and is sufficient to increase gene expression. Furthermore, ectopic overexpression of c-Jun renders breast cancer cells dependent on GLS activity. These findings reveal a role for c-Jun as a driver of cancer cell metabolic reprogramming, and suggest that cancers overexpressing JUN may be especially sensitive to GLS-targeted therapies. The onset of proliferation imposes a range of biosynthetic and bioenergetic demands on mammalian cells, which are met by a fundamental reprogramming of cellular metabolism [1] , [2] . The metabolic phenotype of proliferating cells, including cancer cells, typically includes high rates of glucose uptake and glycolysis coupled to lactate secretion (the Warburg effect) [3] , elevated de novo nucleotide biosynthesis [4] , and a high flux of mitochondrial glutamine oxidation [5] , [6] , [7] . Increased nutrient uptake and re-routing of metabolites into anabolic processes are not passive adaptations to the proliferative state, but instead are tightly regulated by the signal transduction pathways and transcriptional networks that promote cell growth and cell cycle progression. Thus, many of the oncogenic signals that lead to cellular transformation directly impact cancer cell metabolism [8] . Metabolic reprogramming supports the proliferative state but can render cancer cells ‘addicted’ to certain nutrients, and therefore provides opportunities for novel therapeutic interventions [9] . Some cancer cells show an absolute requirement for an exogenous supply of glutamine, the most abundant amino acid in plasma. Glutamine has many metabolic fates inside the cell, acting as a carbon and nitrogen source for biosynthetic reactions and also contributing to redox homoeostasis [5] , [6] , [7] . However, it is the role of glutamine as an anaplerotic substrate for the tricarboxylic acid (TCA) cycle that underlies the ‘glutamine addiction’ of many rapidly proliferating cells [10] , [11] . The sequential conversion of glutamine to glutamate, and then to the TCA cycle intermediate α-ketoglutarate (α-KG), provides a mechanism for replenishing carbon that is lost from the cycle to anabolic pathways. The first reaction is catalysed by the mitochondrial enzyme glutaminase (GLS), and the second reaction by glutamate dehydrogenase or by one of several transaminase enzymes. Two genes, GLS and GLS2 , encode glutaminase enzymes in mammals [12] . The GLS gene encodes two splice variants, referred to as kidney-type glutaminase and glutaminase C (GAC), while the GLS2 gene encodes two proteins through a surrogate promoter mechanism, liver-type glutaminase and GAB [12] . Whereas the GLS2 isozymes are downregulated in several cancers [13] , the GLS isozymes, in particular the GAC splice variant, are frequently upregulated in cancers of the breast [14] , lung [15] , colon [16] , prostate [17] and brain [18] . Recently, two classes of small-molecule inhibitors of GLS have been identified, based on the lead compounds bis-2-(5-phenylacetamido-1,2,4-thiadiazol-2-yl)ethyl sulfide (BPTES) and 968 (refs 19 , 20 ). Inhibition of GLS by these molecules, or siRNA-mediated knockdown of GLS, severely impacts the proliferation and/or survival of several cancer cell lines, but does not appear to have detrimental effects on non-tumorigenic cells [20] , [21] . Thus, there is considerable interest in targeting GLS as a therapeutic strategy against cancer, and the BPTES derivative CB-839 is currently undergoing clinical trials [21] . One regulator of GLS expression and glutamine catabolism is the transcription factor c-Myc [22] , [23] . In P493 Burkitt’s lymphoma and PC3 prostate cancer cell lines, c-Myc upregulates GLS through an indirect mechanism involving transcriptional repression of micro-RNAs miR-23a/b, which target the 3′-UTR of the GLS transcript and suppress its translation [23] . However, the relationship between c-Myc and glutamine metabolism is complex and tissue specific [24] , and tumour-specific alternative polyadenylation of the GLS transcript can cause a switch of the 3′-UTR, allowing it to escape c-Myc/miR-23-mediated regulation [25] . An apparent uncoupling of c-Myc and GLS has recently been described in human mammary epithelial cells as well as in certain breast cancer cell lines [26] , [27] . We previously reported that mitochondrial glutaminase activity becomes elevated during Rho GTPase-mediated cellular transformation [20] . Here we show that the oncogenic transcription factor c-Jun is essential for this signalling outcome, and also acts as a primary regulator of GLS expression in human breast cancer cells. Moreover, we demonstrate that overexpression of the JUN proto-oncogene is sufficient to sensitize breast cancer cells to glutaminase-targeted therapy. Rho GTPases can drive glutamine-dependent transformation We previously reported that oncogenic-Dbl, a guanine nucleotide exchange factor and potent activator of Rho GTPases, signals to upregulate mitochondrial GLS activity in NIH/3T3 cells [20] . This is an essential event for maintaining Dbl-induced cellular transformation. To explore further the signalling connections that link Rho GTPases with GLS, we utilized an inducible, tetracycline-off, system to control the expression of oncogenic-Dbl in mouse embryonic fibroblasts (MEFs). When doxycycline (0.6 μg ml −1 ) is present in the culture medium, HA-tagged oncogenic-Dbl is undetectable by western blot analysis of whole-cell lysates. Removal of doxycycline triggers a robust expression of oncogenic-Dbl within 10 h that remains elevated through 72 h ( Fig. 1a ). This is accompanied by a corresponding increase in GLS protein levels, which peak 24–48 h following induction ( Fig. 1a ). We isolated mitochondria from uninduced and induced MEFs and assayed the preparations for glutaminase activity as described previously [28] . This confirmed that induction of oncogenic-Dbl results in elevated glutaminase activity ( Fig. 1b ). We then tested whether GLS was upregulated at the transcriptional level. Cells that were either uninduced or induced (24 h) were analysed by real-time PCR (RT–PCR), which revealed that induction of oncogenic-Dbl expression leads to an ∼ 12-fold increase of the GLS transcript ( Fig. 1c ). 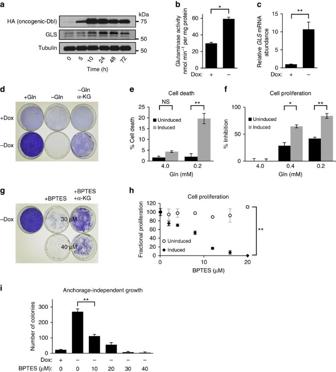Figure 1: Glutamine-dependent transformation by oncogenic-Dbl. (a) Western blot analysis showing timecourse of oncogenic-Dbl expression in an inducible MEF system, and downstream elevation of GLS levels. Cells were induced by plating in doxycycline-free growth medium, and samples were collected at time-points up to 72 h. (b) Glutaminase activity assay using mitochondria isolated from MEFs in which oncogenic-Dbl expression was either uninduced (+Dox) or induced for 24 h (−Dox). Activity is expressed per mg of total cellular protein, and data presented are the mean±s.d. of triplicate assays. (c) RT–PCR analysis of uninduced and induced (24 h) MEFs, showing relative levels of theGLStranscript. The data presented are the RQ values, with error bars marking RQ max and RQ min, from triplicate reactions. (d) Saturation density analysis showing the effect of glutamine withdrawal on oncogenic-Dbl inducible MEFs. Dishes of uninduced (+Dox) and induced (−Dox) cells cultured in 4 mM glutamine, or in glutamine-free medium ±2 mM dimethyl α-ketoglutarate, were fixed and then stained with crystal violet. (e) Cell death analysis for uninduced or induced cells after 6 days culture in 4.0 or 0.2 mM glutamine. Data presented are the mean±s.d. of triplicate assays. (f) Cell proliferation assays showing the effect of glutamine depletion on proliferation of uninduced and induced MEFs over 6 days. Data presented are the mean±s.d. of triplicate assays. (g) Saturation density analysis showing the effect of the GLS inhibitor BPTES on oncogenic-Dbl induced MEFs. Induced (−Dox) cells cultured in the absence or presence of BPTES (30 or 40 μM)±2 mM dimethyl α-ketoglutarate were fixed and then stained with crystal violet. (h) BPTES dose curves showing the effect of different BPTES concentrations on proliferation over 6 days of uninduced or induced MEFs. Fractional proliferation relative to untreated cells is shown. Assays were carried out in 10% FBS medium, and data presented are the mean±s.d. of triplicate assays. (i) Anchorage-independent growth assay for uninduced (+Dox) cells, and for induced (−Dox) cells cultured under increasing BPTES concentrations. Data presented are the mean±s.d. of triplicate assays. Differences were analysed with Student’st-test. *P<0.05, **P<0.01. Figure 1: Glutamine-dependent transformation by oncogenic-Dbl. ( a ) Western blot analysis showing timecourse of oncogenic-Dbl expression in an inducible MEF system, and downstream elevation of GLS levels. Cells were induced by plating in doxycycline-free growth medium, and samples were collected at time-points up to 72 h. ( b ) Glutaminase activity assay using mitochondria isolated from MEFs in which oncogenic-Dbl expression was either uninduced (+Dox) or induced for 24 h (−Dox). Activity is expressed per mg of total cellular protein, and data presented are the mean±s.d. of triplicate assays. ( c ) RT–PCR analysis of uninduced and induced (24 h) MEFs, showing relative levels of the GLS transcript. The data presented are the RQ values, with error bars marking RQ max and RQ min, from triplicate reactions. ( d ) Saturation density analysis showing the effect of glutamine withdrawal on oncogenic-Dbl inducible MEFs. Dishes of uninduced (+Dox) and induced (−Dox) cells cultured in 4 mM glutamine, or in glutamine-free medium ±2 mM dimethyl α-ketoglutarate, were fixed and then stained with crystal violet. ( e ) Cell death analysis for uninduced or induced cells after 6 days culture in 4.0 or 0.2 mM glutamine. Data presented are the mean±s.d. of triplicate assays. ( f ) Cell proliferation assays showing the effect of glutamine depletion on proliferation of uninduced and induced MEFs over 6 days. Data presented are the mean±s.d. of triplicate assays. ( g ) Saturation density analysis showing the effect of the GLS inhibitor BPTES on oncogenic-Dbl induced MEFs. Induced (−Dox) cells cultured in the absence or presence of BPTES (30 or 40 μM)±2 mM dimethyl α-ketoglutarate were fixed and then stained with crystal violet. ( h ) BPTES dose curves showing the effect of different BPTES concentrations on proliferation over 6 days of uninduced or induced MEFs. Fractional proliferation relative to untreated cells is shown. Assays were carried out in 10% FBS medium, and data presented are the mean±s.d. of triplicate assays. ( i ) Anchorage-independent growth assay for uninduced (+Dox) cells, and for induced (−Dox) cells cultured under increasing BPTES concentrations. Data presented are the mean±s.d. of triplicate assays. Differences were analysed with Student’s t -test. * P <0.05, ** P <0.01. Full size image Induction of oncogenic-Dbl caused MEFs to acquire transformed characteristics, including greatly increased saturation density, and the ability to proliferate in low serum (0.5% fetal bovine serum (FBS)) medium and to undergo anchorage-independent growth. Since these changes were accompanied by an increase in GLS levels, we tested whether cellular transformation was dependent on an exogenous supply of glutamine, and/or on GLS enzymatic activity. After 8 days of culture in medium supplemented with 10% FBS±4 mM glutamine, saturation density was assessed by fixing and staining cells with crystal violet ( Fig. 1d ). Prior to fixation, cells were imaged at × 100 magnification ( Supplementary Fig. 1a ). The increased saturation density of cells expressing oncogenic-Dbl was completely abolished in glutamine-free medium, but could be partially rescued by supplementation with a cell-permeable analogue of α-ketoglutarate (dimethyl-α-KG), a downstream metabolite of the GLS reaction. We compared cell viability under high-glutamine (4 mM) and low-glutamine (0.2 mM) conditions, and found that uninduced cells remained fully viable following glutamine depletion, whereas induced cells showed an ∼ 5-fold increase in cell death ( Fig. 1e ). The proliferation rate of both uninduced and induced cells decreased on glutamine deprivation, although the inhibition was ∼ 2-fold greater in induced cells ( Fig. 1f ). We then used BPTES [19] , a small-molecule inhibitor of GLS, to test whether MEFs transformed by oncogenic-Dbl were dependent on GLS activity. Saturation density of induced cells was decreased by BPTES treatment in a dose-dependent manner, and partially rescued by supplementation with dimethyl-α-KG ( Fig. 1g and Supplementary Fig. 1b ). Cell proliferation assays illustrated the remarkable difference in BPTES sensitivity between uninduced and induced MEFs ( Fig. 1h ). Proliferation of induced cells was potently inhibited by BPTES with an IC 50 of 8 μM, whereas uninduced cells were unaffected even by 20 μM BPTES. Oncogenic-Dbl-induced cells, but not uninduced cells, were capable of anchorage-independent growth. This too was completely blocked by BPTES treatment ( Fig. 1i ). Rho GTPases signal to c-Jun to upregulate GLS expression The results above show that oncogenic-Dbl signals to upregulate GLS at the transcript and protein level, and that cellular transformation driven by oncogenic-Dbl is dependent on GLS activity and an exogenous supply of glutamine. We next wanted to identify the signalling pathway downstream of the Rho GTPases that was responsible for regulating GLS expression. We first used phospho-specific antibodies to assess the effects of oncogenic-Dbl induction on key cellular signalling proteins. Here, and throughout the study, low-serum conditions (0.5% FBS) were used for signalling experiments to minimize ‘background’ cellular signalling activity. Western blot analysis of whole-cell lysates revealed an extremely potent activation of the MKK4/c-Jun N-terminal kinase (JNK) signalling axis on induction (24 h), and downstream activating phosphorylation of the oncogenic transcription factor c-Jun ( Fig. 2a ). c-Jun is known to autoregulate its own gene expression in MEFs [29] , [30] and, consistent with this, we found that total c-Jun levels increased as well as phosphorylated c-Jun levels (2-fold and 26-fold, respectively) ( Fig. 2a and Supplementary Fig. 2a ). The JNK kinase MKK7 and the Jun-family members JunB and JunD were expressed at low levels, and phosphorylated forms could not be detected ( Supplementary Fig. 2b,c ). Another target of MKK4, p38, was phosphorylated downstream of oncogenic-Dbl, whereas the activation status of ERK showed only a subtle change ( Fig. 2b ). Rho-associated coiled-coil containing protein kinase (ROCK) was likely activated, as indicated by increased phosphorylation of its substrate myosin light chain 2 (MLC 2) ( Fig. 2c ). Consistent with earlier reports that ROCK signals to inhibit Akt [31] , a modest decrease in Akt phosphorylation at residue T308 occurred on induction ( Fig. 2d ), and this could be rescued by inhibition of ROCK ( Supplementary Fig. 2d ). The mTORC1-S6K signalling axis showed little change on oncogenic-Dbl induction, and we also detected no change in the phosphorylation level of AMPKα ( Fig. 2d ). 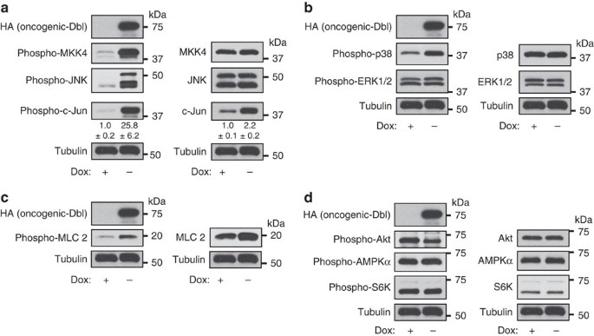Figure 2: Oncogenic-Dbl potently activates the MKK4-JNK-c-Jun signalling axis in MEFs. Western blot analysis of whole-cell lysates of MEFs in which oncogenic-Dbl expression was either uninduced (+Dox) or induced for 24 h (−Dox) under low-serum (0.5% FBS) conditions. The extent of activation of different signalling pathways was assessed using phospho-specific antibodies that recognize activated kinases or their downstream phosphorylation targets (left panels). Any changes in total protein levels were also assessed (right panels). (a) The MAPK signalling axis involving MKK4-JNK-c-Jun is potently activated downstream of oncogenic-Dbl. Total c-Jun levels are also elevated, consistent with previous reports showing auto-regulation ofJUNexpression. (b) The MAPK p38 is moderately activated, whereas ERK is only slightly activated on oncogenic-Dbl induction. (c) ROCK activity, as read-out by MLC 2 phosphorylation, is activated on induction. (d) Akt is slightly inhibited, and AMPK and mTORC1 activity (the latter read-out by S6K phosphorylation) are largely unaffected by oncogenic-Dbl induction. Relative densitometry data are the mean±s.d. of triplicate blots. Figure 2: Oncogenic-Dbl potently activates the MKK4-JNK-c-Jun signalling axis in MEFs. Western blot analysis of whole-cell lysates of MEFs in which oncogenic-Dbl expression was either uninduced (+Dox) or induced for 24 h (−Dox) under low-serum (0.5% FBS) conditions. The extent of activation of different signalling pathways was assessed using phospho-specific antibodies that recognize activated kinases or their downstream phosphorylation targets (left panels). Any changes in total protein levels were also assessed (right panels). ( a ) The MAPK signalling axis involving MKK4-JNK-c-Jun is potently activated downstream of oncogenic-Dbl. Total c-Jun levels are also elevated, consistent with previous reports showing auto-regulation of JUN expression. ( b ) The MAPK p38 is moderately activated, whereas ERK is only slightly activated on oncogenic-Dbl induction. ( c ) ROCK activity, as read-out by MLC 2 phosphorylation, is activated on induction. ( d ) Akt is slightly inhibited, and AMPK and mTORC1 activity (the latter read-out by S6K phosphorylation) are largely unaffected by oncogenic-Dbl induction. Relative densitometry data are the mean±s.d. of triplicate blots. Full size image Since ROCK, p38 and JNK signalling were all activated downstream of oncogenic-Dbl, we tested whether selective inhibition of these kinases (by the small-molecule inhibitors Y-27632, SB203580 and SP600125, respectively) impacted the ability of oncogenic-Dbl to upregulate GLS. Cells were induced for 48 h, either in the absence or presence of 10 μM of each inhibitor, and whole-cell lysates were then analysed by western blot. Treatment of induced cells with the ROCK inhibitor Y-27632 or the p38 inhibitor SB203580 did not significantly impact GLS levels, whereas the JNK inhibitor SP600125 largely blocked the upregulation of GLS ( Fig. 3a ). Although rapamycin-sensitive mTORC1 can influence GLS levels by increasing MYC translation [32] , we found that regulation of GLS downstream of the Rho GTPases was independent of mTORC1 activity ( Fig. 3b ), and changes in c-Myc (and phospho-c-Myc) levels did not fully correspond to changes in GLS ( Supplementary Fig. 2e ). Treatment of induced cells with the c-Myc inhibitor 10058-F4 severely impacted viability in low-serum (0.5% FBS) culture medium (no viable cells remained after 24 h treatment with 10 μM 10058-F4), and it is possible that c-Myc contributes to the regulation of GLS expression by Rho GTPases under these conditions. In high-serum (10% FBS) medium, treatment with 10058-F4 at concentrations up to 60 μM had little impact on GLS levels in induced cells ( Supplementary Fig. 2f ), whereas inhibition of JNK by 10 μM SP600125 still suppressed GLS expression ( Supplementary Fig. 2e ). 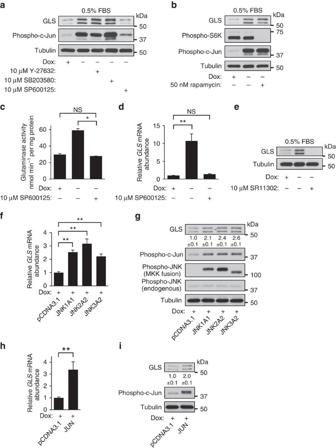Figure 3: Oncogenic-Dbl signals to c-Jun to upregulate GLS in MEFs. (a) Western blot analysis of whole-cell lysates of uninduced (+Dox) or induced for 48 h (−Dox) MEFs±10 μM selective inhibitors of ROCK (Y-27632), p38 (SB203580) or JNK (SP600125). Inhibition of JNK largely blocks the upregulation of GLS downstream of oncogenic-Dbl. (b) Western blot analysis showing that inhibition of mTORC1 by rapamycin has little effect on the upregulation of GLS downstream of oncogenic-Dbl. (c) Glutaminase activity assay using mitochondria isolated from uninduced (+Dox) MEFs and from MEFs that had been induced for 24 h (−Dox) in the absence or presence of 10 μM SP600125 (JNK inhibitor). Activity is expressed per mg of total cellular protein and data presented are the mean±s.d. of triplicate assays. (d) RT–PCR analysis of uninduced (+Dox) and 24 h induced (−Dox) MEFs±10 μM SP600125, showing relative levels of theGLStranscript. The data presented are the RQ values, with error bars marking RQ max and RQ min, from triplicate reactions. (e) Western blot analysis showing that the AP-1 inhibitor SR11302 (10 μM) completely blocksGLSexpression in oncogenic-Dbl-induced MEFs. (f) RT–PCR analysis showing that transient transfection of uninduced (+Dox) MEFs with constitutively activated JNK/MKK fusion constructs leads to increasedGLSmRNA abundance. The data presented are the RQ values, with error bars marking RQ max and RQ min, from triplicate reactions. (g) Western blot analysis of the samples from the previous panel, showing that ectopic expression of constitutively activated JNK fusion constructs in uninduced MEFs leads to increased phosphorylation of c-Jun and upregulated GLS protein levels. (h) RT–PCR analysis showing that transient transfection of uninduced (+Dox) MEFs with a construct for expressing theJUNproto-oncogene leads to increasedGLSmRNA abundance. The data presented are the RQ values, with error bars marking RQ max and RQ min, from triplicate reactions. (i) Western blot analysis of the samples from the previous panel, showing that ectopic expression ofJUNin uninduced MEFs leads to increased levels of phospho-c-Jun and upregulated GLS protein levels. Note that the ectopically expressed c-Jun contains a V5-tag, and consequently runs at a slightly higher molecular weight than endogenous c-Jun. Relative densitometry data are the mean±s.d. of triplicate blots. Differences were analysed with Student’st-test. *P<0.05, **P<0.01. Figure 3: Oncogenic-Dbl signals to c-Jun to upregulate GLS in MEFs. ( a ) Western blot analysis of whole-cell lysates of uninduced (+Dox) or induced for 48 h (−Dox) MEFs±10 μM selective inhibitors of ROCK (Y-27632), p38 (SB203580) or JNK (SP600125). Inhibition of JNK largely blocks the upregulation of GLS downstream of oncogenic-Dbl. ( b ) Western blot analysis showing that inhibition of mTORC1 by rapamycin has little effect on the upregulation of GLS downstream of oncogenic-Dbl. ( c ) Glutaminase activity assay using mitochondria isolated from uninduced (+Dox) MEFs and from MEFs that had been induced for 24 h (−Dox) in the absence or presence of 10 μM SP600125 (JNK inhibitor). Activity is expressed per mg of total cellular protein and data presented are the mean±s.d. of triplicate assays. ( d ) RT–PCR analysis of uninduced (+Dox) and 24 h induced (−Dox) MEFs±10 μM SP600125, showing relative levels of the GLS transcript. The data presented are the RQ values, with error bars marking RQ max and RQ min, from triplicate reactions. ( e ) Western blot analysis showing that the AP-1 inhibitor SR11302 (10 μM) completely blocks GLS expression in oncogenic-Dbl-induced MEFs. ( f ) RT–PCR analysis showing that transient transfection of uninduced (+Dox) MEFs with constitutively activated JNK/MKK fusion constructs leads to increased GLS mRNA abundance. The data presented are the RQ values, with error bars marking RQ max and RQ min, from triplicate reactions. ( g ) Western blot analysis of the samples from the previous panel, showing that ectopic expression of constitutively activated JNK fusion constructs in uninduced MEFs leads to increased phosphorylation of c-Jun and upregulated GLS protein levels. ( h ) RT–PCR analysis showing that transient transfection of uninduced (+Dox) MEFs with a construct for expressing the JUN proto-oncogene leads to increased GLS mRNA abundance. The data presented are the RQ values, with error bars marking RQ max and RQ min, from triplicate reactions. ( i ) Western blot analysis of the samples from the previous panel, showing that ectopic expression of JUN in uninduced MEFs leads to increased levels of phospho-c-Jun and upregulated GLS protein levels. Note that the ectopically expressed c-Jun contains a V5-tag, and consequently runs at a slightly higher molecular weight than endogenous c-Jun. Relative densitometry data are the mean±s.d. of triplicate blots. Differences were analysed with Student’s t -test. * P <0.05, ** P <0.01. Full size image Consistent with the effects on GLS protein levels, treatment with the JNK inhibitor SP600125 (10 μM) completely blocked the increase in mitochondrial glutaminase activity that occurs downstream of oncogenic-Dbl signalling ( Fig. 3c ). Because JNK directly phosphorylates activator protein 1 (AP-1) family transcription factors including the archetypal substrate c-Jun, leading to increased transcriptional activity, we tested whether blockade of JNK signalling affected GLS transcript levels. The ∼ 12-fold increase in GLS mRNA that occurs following oncogenic-Dbl induction was completely abolished by 10 μM SP600125 ( Fig. 3d ). To test the hypothesis that the effects of JNK inhibition were mediated by suppression of c-Jun transcriptional activity, we treated induced cells with 10 μM SR11302, a selective inhibitor of the AP-1 family of transcription factors to which c-Jun belongs [33] . This resulted in the complete loss of GLS to undetectable levels ( Fig. 3e ). The experiments above suggested that the signal to elevate GLS expression downstream of oncogenic-Dbl is transmitted via JNK-mediated phosphorylation of a Jun-family AP-1 transcription factor, most likely c-Jun, since it is highly expressed in these cells ( Fig. 2a ), in contrast to JunB and JunD (Supplementary Fig. 2c). To test whether JNK and c-Jun can upregulate GLS expression, we transiently transfected uninduced MEFs with constructs for expressing constitutively activated MKK/JNK fusion proteins [34] or c-Jun. Uninduced cells were cultured for 48 h after transfection (in 10% FBS medium, as transfection reagents harmed viability of MEFs in 0.5% FBS medium), and then analysed by RT–PCR and western blot. Ectopic expression of JNK1, JNK2 or JNK3 fusion-constructs all led to elevated GLS transcript levels relative to vector-control cells ( Fig. 3f ). Western blot analyses of whole-cell lysates showed that phospho-c-Jun and GLS were both elevated downstream of the JNK constructs ( Fig. 3g ). Similarly, ectopic expression of the JUN gene resulted in upregulated GLS transcript levels ( Fig. 3h ), and elevated levels of both phospho-c-Jun and GLS ( Fig. 3i ). Collectively, these results indicate that, downstream of oncogenic Rho GTPase signalling, JNK transmits a signal to increase transcription of the GLS gene by phosphorylating and activating the oncogenic transcription factor c-Jun. This prompted us to investigate the possible role of c-Jun in regulating GLS expression in human cancer cells. c-Jun and GLS correlate in human breast cancer cell lines Because the JUN proto-oncogene is overexpressed, and associated with aggressive behaviour, in a subset of human breast cancers [35] , [36] , [37] , we probed a panel of 12 breast cancer cell lines for c-Jun and GLS. First, we obtained an estimate of the glutamine dependence of each cell line by assaying proliferation over 6 days in culture medium containing either 2.0 or 0.1 mM glutamine ( Supplementary Fig. 3 ). We then collected cells at ∼ 60% confluency from complete RPMI medium (10% FBS, 2 mM glutamine) and probed whole-cell lysates by western blot, with samples ordered by increasing glutamine dependence of the cell line, left to right. This revealed a very strong correlation ( R =0.85) between relative levels of c-Jun and GLS ( Fig. 4a and Supplementary Fig. 4a ). In particular, cell lines with high endogenous c-Jun levels (BT-549, Hs 578T, MDA-MB-231 and TSE) all showed highly elevated GLS levels. The level of c-Jun also correlated very strongly with the glutamine dependence of the cell lines ( R =0.83; see Supplementary Fig. 4b ) and moderately strongly with their proliferation rates ( R =0.63; see Supplementary Fig. 4c ). The abundance of activated c-Jun, as indicated by phosphorylation at residue S73 (a JNK target residue), similarly correlated very strongly with GLS ( Fig. 4a ), whereas the related Jun-family transcription factors, JunB and JunD, showed less correlation ( Fig. 4b ). Relative levels of glutamate dehydrogenase (GLUD1/2) showed little variation among the cell lines ( Supplementary Fig. 5 ). 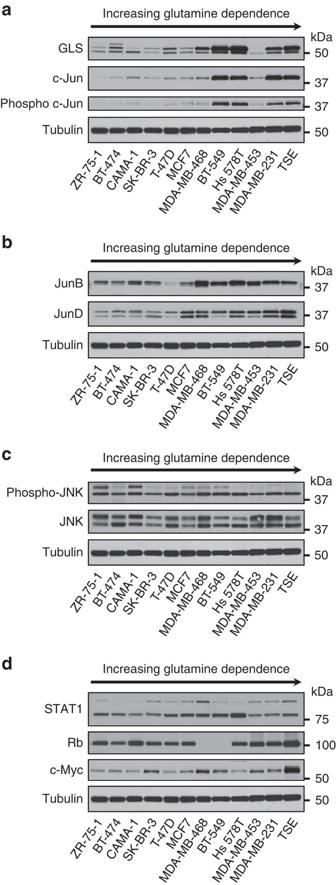Figure 4: c-Jun correlates strongly with GLS levels in human breast cancer cell lines. Cells were collected at∼60% confluency from RPMI growth medium supplemented with 10% FBS, and whole-cell lysates prepared and analysed by western blot. Samples were ordered according to glutamine dependence, increasing from left to right (Supplementary Fig. 3). (a) Correlation between c-Jun/phospho-c-Jun and GLS levels. Quantification of GLS and c-Jun band intensities allowed a Pearson correlation coefficient of 0.85 to be determined (Supplementary Fig. 4a). (b) Other Jun-family members do not correlate strongly with GLS levels. (c) Under 10% FBS culture conditions, p46 JNK (lower band) is active in all of the breast cancer cell lines. Neither JNK nor phospho-JNK correlate with GLS levels. (d) Other reported regulators ofGLSexpression do not strongly correlate with GLS levels. Figure 4: c-Jun correlates strongly with GLS levels in human breast cancer cell lines. Cells were collected at ∼ 60% confluency from RPMI growth medium supplemented with 10% FBS, and whole-cell lysates prepared and analysed by western blot. Samples were ordered according to glutamine dependence, increasing from left to right ( Supplementary Fig. 3 ). ( a ) Correlation between c-Jun/phospho-c-Jun and GLS levels. Quantification of GLS and c-Jun band intensities allowed a Pearson correlation coefficient of 0.85 to be determined ( Supplementary Fig. 4a ). ( b ) Other Jun-family members do not correlate strongly with GLS levels. ( c ) Under 10% FBS culture conditions, p46 JNK (lower band) is active in all of the breast cancer cell lines. Neither JNK nor phospho-JNK correlate with GLS levels. ( d ) Other reported regulators of GLS expression do not strongly correlate with GLS levels. Full size image The JNK1 and JNK2 proteins each exist as two splice variants, p46 (predominantly JNK1) and p54 (predominantly JNK2) [30] , [38] , [39] . Whereas p46 JNK1 is the primary kinase for activating c-Jun, endogenous p54 JNK2 can negatively regulate c-Jun stability [30] . We found that p46 JNK is expressed and phosphorylated to a similar extent across the panel of breast cancer cell lines ( Fig. 4c ). In contrast, although p54 JNK is expressed in all cell lines, it only shows strong phosphorylation in ZR-75-1 and CAMA-1 ( Fig. 4c ). Given that p46 JNK is activated in all cell lines, and that phosphorylated c-Jun is proportional to total c-Jun across the panel ( Fig. 4a ), we conclude that differences in total c-Jun activity between the cell lines are due primarily to variations in c-Jun protein levels, rather than to differences in JNK activity. We also probed lysates for three previously reported regulators of GLS, namely c-Myc and STAT1 that upregulate GLS [22] , [23] , [40] , and the retinoblastoma protein (Rb), loss of which leads to elevated GLS levels through an unknown mechanism [41] ( Fig. 4d ). None of these proteins correlated with GLS, although we note that all three are subject to post-translational regulation. The GLS promoter directly binds c-Jun at a consensus motif We next examined whether c-Jun binds directly to the GLS promoter. The promoter region for the human GLS gene was analysed to position −5,000 bp relative to the transcription start site (TSS), and a number of putative c-Jun binding sites (<15% dissimilarity to the consensus sequence) were identified using the PROMO [42] resource ( Supplementary Fig. 6 ). An earlier genome-wide survey of c-Jun binding sites found them to be located in close proximity to the TSS, and mammalian transcription factor binding sites in general are strongly enriched around −200 bp from the TSS [35] , [43] . We found a close match to the consensus c-Jun binding motif (TGA[G/C]TCA) at position −188 bp relative to the TSS of human GLS (5′-TGACTCC-3′) ( Supplementary Figs 6 and 7a ). A close match to the c-Jun consensus motif is also present at position −200 bp in the mouse GLS promoter (5′-TGACACA-3′) ( Supplementary Fig. 7b ). Exact matches to the c-Jun consensus motif (5′-TGAGTCA-3′) were also found at position −2,211 bp for human GLS , and positions −2,469 and −1,545 bp for mouse GLS . We then carried out chromatin immunoprecipitations (ChIPs) to test whether c-Jun binds directly to the GLS promoter. For these experiments, we used MDA-MB-231 breast cancer cells, which have high endogenous levels of both GLS and c-Jun ( Fig. 4a ). Briefly, cross-linked chromatin was digested to a length of ∼ 150–900 bp, and an antibody against endogenous c-Jun was used to immunoprecipitate c-Jun/DNA complexes. A parallel immunoprecipitation was carried out using IgG, as a negative control. Protein-DNA cross-links were then reversed, and RT–PCR was performed using primers designed to amplify a 196-bp fragment centred on the putative c-Jun binding site at position −188 bp relative to the TSS ( Supplementary Fig. 7a ). This yielded a strong signal from the c-Jun ChIP relative to the IgG ChIP, indicating that c-Jun binds to this region of the GLS promoter ( Fig. 5a ). Similar results were obtained using two additional sets of primers to amplify slightly shorter fragments also centred on the predicted c-Jun binding site ( Supplementary Fig. 8 ). 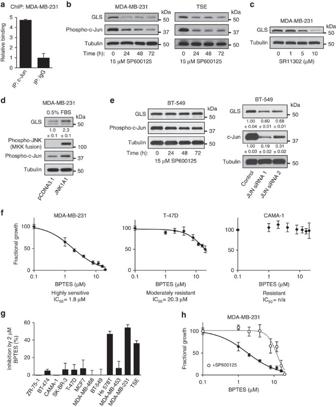Figure 5: Inhibition of c-Jun suppressesGLSexpression and BPTES sensitivity in human breast cancer cell lines. (a) ChIP analysis showing that c-Jun binds to theGLSpromoter. Complexes containing c-Jun were immunoprecipitated from cross-linked, digested, chromatin isolated from MDA-MB-231 cells. A parallel immunoprecipitation using rabbit IgG was carried out as a negative control. Following reversal of cross-links and purification of DNA, RT–PCR was run using primers designed to amplify a 196-bp fragment centred on the putative c-Jun binding site at position −188 bp relative to the TSS. The data presented are the RQ values, with error bars marking RQ max and RQ min, from triplicate reactions. (b) Western blot analysis showing that treatment of MDA-MB-231 or TSE cells with the JNK inhibitor SP600125 (15 μM) leads to decreased phosphorylation of c-Jun, and decreased GLS levels. (c) Treatment of MDA-MB-231 cells with the AP-1 inhibitor SR11302 (1–10 μM) for 48 h results in a dose-dependent decrease in GLS. (d) Western blot analysis showing that transient transfection of MDA-MB-231 cells with a constitutively activated JNK fusion construct results in increased c-Jun phosphorylation and upregulated GLS levels. Cells were collected 48 h after transfection. (e) Western blot analysis showing that in the drug-resistant breast cancer cell line BT-549, treatment with 15 μM SP600125 has little effect on c-Jun phosphorylation and does not lead to decreased GLS levels (left panels). However, knockdown ofJUNexpression using siRNAs leads to decreased GLS levels. Relative band intensities are indicated. (f) Representative BPTES dose curves showing the effect of BPTES on the proliferation of breast cancer cell lines over 6 days. Curves were fitted using SigmaPlot, with data from triplicate assays. (g) Sensitivity of breast cancer cell lines to GLS inhibition, as indicated by inhibition of proliferation over 6 days by 2 μM BPTES. Of the high-c-Jun lines, only the drug-resistant BT-549 cells were not highly sensitive to BPTES. None of the low-c-Jun lines were highly sensitive. Data presented are the mean±s.d. of triplicate assays. (h) BPTES dose curves for MDA-MB-231 cells±15 μM SP600125, showing that inhibition of JNK desensitizes cells to GLS inhibition (the IC50for BPTES shifts from 1.8 to 12 μM). Curves were fitted using SigmaPlot, with data from triplicate assays. Relative densitometry data are the mean±s.d. of triplicate blots. Figure 5: Inhibition of c-Jun suppresses GLS expression and BPTES sensitivity in human breast cancer cell lines. ( a ) ChIP analysis showing that c-Jun binds to the GLS promoter. Complexes containing c-Jun were immunoprecipitated from cross-linked, digested, chromatin isolated from MDA-MB-231 cells. A parallel immunoprecipitation using rabbit IgG was carried out as a negative control. Following reversal of cross-links and purification of DNA, RT–PCR was run using primers designed to amplify a 196-bp fragment centred on the putative c-Jun binding site at position −188 bp relative to the TSS. The data presented are the RQ values, with error bars marking RQ max and RQ min, from triplicate reactions. ( b ) Western blot analysis showing that treatment of MDA-MB-231 or TSE cells with the JNK inhibitor SP600125 (15 μM) leads to decreased phosphorylation of c-Jun, and decreased GLS levels. ( c ) Treatment of MDA-MB-231 cells with the AP-1 inhibitor SR11302 (1–10 μM) for 48 h results in a dose-dependent decrease in GLS. ( d ) Western blot analysis showing that transient transfection of MDA-MB-231 cells with a constitutively activated JNK fusion construct results in increased c-Jun phosphorylation and upregulated GLS levels. Cells were collected 48 h after transfection. ( e ) Western blot analysis showing that in the drug-resistant breast cancer cell line BT-549, treatment with 15 μM SP600125 has little effect on c-Jun phosphorylation and does not lead to decreased GLS levels (left panels). However, knockdown of JUN expression using siRNAs leads to decreased GLS levels. Relative band intensities are indicated. ( f ) Representative BPTES dose curves showing the effect of BPTES on the proliferation of breast cancer cell lines over 6 days. Curves were fitted using SigmaPlot, with data from triplicate assays. ( g ) Sensitivity of breast cancer cell lines to GLS inhibition, as indicated by inhibition of proliferation over 6 days by 2 μM BPTES. Of the high-c-Jun lines, only the drug-resistant BT-549 cells were not highly sensitive to BPTES. None of the low-c-Jun lines were highly sensitive. Data presented are the mean±s.d. of triplicate assays. ( h ) BPTES dose curves for MDA-MB-231 cells±15 μM SP600125, showing that inhibition of JNK desensitizes cells to GLS inhibition (the IC 50 for BPTES shifts from 1.8 to 12 μM). Curves were fitted using SigmaPlot, with data from triplicate assays. Relative densitometry data are the mean±s.d. of triplicate blots. Full size image c-Jun regulates GLS expression and BPTES sensitivity Since c-Jun directly binds the promoter of the GLS gene, and endogenous levels of c-Jun and GLS correlate strongly in human breast cancer cell lines, we determined whether inhibition of JNK, inhibition of AP-1 family transcription factors, or knockdowns of c-Jun, affected GLS levels in these cells. We first inhibited JNK using 15 μM SP600125 in the high-GLS cell lines MDA-MB-231 and TSE. This led to a sharp decrease in phospho-c-Jun levels, and GLS expression was strongly suppressed within 24 h and remained so through 72 h ( Fig. 5b ). We also directly inhibited AP-1 transcriptional activity in MDA-MB-231 cells using SR11302 (48 h), and observed a dose-dependent suppression of GLS expression ( Fig. 5c ). Reciprocally, ectopic expression of a constitutively activated JNK1 fusion protein in MDA-MB-231 cells, under low serum (0.5% FBS) conditions, resulted in elevated c-Jun phosphorylation and elevated GLS levels ( Fig. 5d ). In BT-549 cells, which are reported to be relatively drug-resistant [44] , treatment with 15 μM SP600125 caused only a very modest inhibition of c-Jun phosphorylation ( Fig. 5e , left panel). Consistent with this, SP600125 treatment did not lead to decreased GLS levels in this cell line, and we therefore used siRNAs to knockdown JUN expression. Prolonged depletion of c-Jun in BT-549 cells (and in other cell lines with high endogenous c-Jun levels) could not be tolerated and resulted in cell death. Nevertheless, whole-cell lysates from BT-549 cells treated with JUN -targeted siRNAs and collected after 48 h repeatedly showed that GLS levels were lower in c-Jun-depleted cells ( Fig. 5e , right panel). Quantification of band intensities confirmed that the degree of c-Jun depletion correlated with the degree of GLS depletion. The results above indicate that the relationship between c-Jun and GLS levels in breast cancer cells is not only correlative but is also causative. We therefore examined whether cell lines with high c-Jun levels are more sensitive to the GLS inhibitor BPTES. Proliferation assays were carried out for all 12 breast cancer cell lines under a range of BPTES concentrations. Defining highly sensitive cell lines as those with an IC 50 <10 μM BPTES, none of the eight cell lines with low c-Jun levels were highly sensitive to BPTES, whereas three of the four cell lines with high c-Jun levels were highly sensitive ( Supplementary Table 1 ). The one exception was the drug-resistant cell line BT-549. Representative dose curves for a highly sensitive cell line (MDA-MB-231, IC 50 =1.8 μM), a moderately resistant cell line (T-47D, IC 50 =20 μM), and a highly resistant cell line (CAMA-1, IC 50 =n/a) are shown ( Fig. 5f ). The much greater BPTES sensitivity of the high c-Jun cell lines, Hs 578T, MDA-MB-231 and TSE, relative to the low c-Jun lines, is illustrated by the response to 2 μM BPTES ( Fig. 5g and Supplementary Fig. 9 ). Inhibition of JNK by SP600125 led to a sharp decrease in GLS levels in MDA-MB-231 (and other) breast cancer cells (see above). We therefore carried out proliferation assays to compare BPTES sensitivity of MDA-MB-231 cells cultured in the absence or presence of 15 μM SP600125. Treatment with the JNK inhibitor sharply decreases the proliferation rate relative to untreated cells. However, the slow proliferation that still occurs in the presence of SP600125 is markedly desensitized to BPTES, with the IC 50 for BPTES shifting ∼ 7-fold from 1.8 to 12 μM ( Fig. 5h ). c-Jun is sufficient to elevate GLS in breast cancer cells Using the MDA-MB-468 breast cancer cell line, which exhibits relatively low endogenous levels of c-Jun and moderate levels of GLS ( Fig. 4a ), we generated derivative cell lines that stably overexpress JUN-V5 or carry the empty plasmid vector. We then collected vector-control cells and JUN -overexpressing cells at ∼ 60% confluency from RPMI medium (10% FBS, 2 mM glutamine), and probed whole-cell lysates for GLS, c-Jun and V5-tag by western blot ( Fig. 6a ). This showed that GLS levels are elevated in the JUN -overexpressing cells relative to the vector-control cells. Mitochondria isolated from the two cell lines were assayed for glutaminase activity, which was markedly higher in the JUN -overexpressing cells ( Fig. 6b ). Moreover, RT–PCR analysis confirmed that GLS transcript levels were upregulated in JUN -overexpressing cells relative to vector-control cells ( Fig. 6c ). We made equivalent derivative cell lines of the MCF7 parental cell line, which has very low endogenous levels of both c-Jun and GLS ( Fig. 4a ), and similarly found that GLS expression was upregulated in JUN -overexpressing cells ( Supplementary Fig. 10a ). 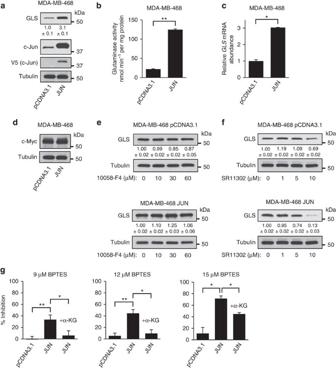Figure 6: c-Jun increasesGLSexpression and BPTES sensitivity in breast cancer cells. (a) Western blot analysis of GLS and c-Jun levels in whole-cell lysates of MDA-MB-468 cells, stably carrying either pCDNA3.1 or theJUN-V5expression vector pCDNA3.1-JUN. Relative band intensities are indicated for GLS. (b) Glutaminase activity assay using mitochondria isolated from the derivative MDA-MB-468 cell lines. Activity is expressed per mg of total cellular protein, and data presented are the mean±s.d. of triplicate assays. (c) RT–PCR analysis of the derivative MDA-MB-468 cell lines, showing relative abundance of theGLStranscript. The data presented are the RQ values, with error bars marking RQ max and RQ min, from triplicate reactions. (d) Western blot analysis showing c-Myc levels in the derivative cell lines. (e) Western blot analysis showing that treatment of vector-control, orJUN-overexpressing, MDA-MB-468 cells with the c-Myc inhibitor 10058-F4 at concentrations up to 60 μM for 48 h has little effect on GLS levels. Relative band intensities are indicated for GLS. (f) Western blot analysis showing that treatment with the AP-1 inhibitor SR11302 (1–10 μM) for 48 h leads to a dose-dependent decrease in GLS levels. The effect is especially pronounced inJUN-overexpressing cells. (g) Cell proliferation assays for MDA-MB-468 cells stably carrying pCDNA3.1 or theJUNexpression vector. Cells were seeded in 12-well dishes at a density of 1 × 104cells per well, cultured for 6 days in the absence or presence of 9 μM (left panel), 12 μM (middle panel) or 15 μM (right panel) BPTES±1 mM dimethyl α-KG. Inhibition of proliferation by BPTES treatment is plotted as a percentage. The data presented are the mean±s.d. of triplicate assays. Relative densitometry data are the mean±s.d. of triplicate blots. Differences were analysed with Student’st-test. *P<0.05,**P<0.01. Figure 6: c-Jun increases GLS expression and BPTES sensitivity in breast cancer cells. ( a ) Western blot analysis of GLS and c-Jun levels in whole-cell lysates of MDA-MB-468 cells, stably carrying either pCDNA3.1 or the JUN-V5 expression vector pCDNA3.1-JUN. Relative band intensities are indicated for GLS. ( b ) Glutaminase activity assay using mitochondria isolated from the derivative MDA-MB-468 cell lines. Activity is expressed per mg of total cellular protein, and data presented are the mean±s.d. of triplicate assays. ( c ) RT–PCR analysis of the derivative MDA-MB-468 cell lines, showing relative abundance of the GLS transcript. The data presented are the RQ values, with error bars marking RQ max and RQ min, from triplicate reactions. ( d ) Western blot analysis showing c-Myc levels in the derivative cell lines. ( e ) Western blot analysis showing that treatment of vector-control, or JUN -overexpressing, MDA-MB-468 cells with the c-Myc inhibitor 10058-F4 at concentrations up to 60 μM for 48 h has little effect on GLS levels. Relative band intensities are indicated for GLS. ( f ) Western blot analysis showing that treatment with the AP-1 inhibitor SR11302 (1–10 μM) for 48 h leads to a dose-dependent decrease in GLS levels. The effect is especially pronounced in JUN -overexpressing cells. ( g ) Cell proliferation assays for MDA-MB-468 cells stably carrying pCDNA3.1 or the JUN expression vector. Cells were seeded in 12-well dishes at a density of 1 × 10 4 cells per well, cultured for 6 days in the absence or presence of 9 μM (left panel), 12 μM (middle panel) or 15 μM (right panel) BPTES±1 mM dimethyl α-KG. Inhibition of proliferation by BPTES treatment is plotted as a percentage. The data presented are the mean±s.d. of triplicate assays. Relative densitometry data are the mean±s.d. of triplicate blots. Differences were analysed with Student’s t -test. * P <0.05, ** P <0.01. Full size image The level of c-Myc did not vary between the vector-control and JUN -overexpressing cells ( Fig. 6d ), and treatment with the c-Myc inhibitor 10058-F4 at concentrations up to 60 μM (48 h) had little effect on GLS levels in the derivative cell lines ( Fig. 6e and Supplementary Fig. 10b ). In contrast, treatment with the AP-1 inhibitor SR11302 (1–10 μM) caused a dose-dependent suppression of GLS in both cell lines, an effect that was especially pronounced in the JUN -overexpressing cells ( Fig. 6f ). Overexpression of JUN sensitizes cancer cells to BPTES As described above, MDA-MB-231 cells treated with the JNK inhibitor SP600125 become desensitized to the GLS inhibitor BPTES ( Fig. 5h ). To complement this result, we carried out proliferation assays to determine whether overexpression of the JUN proto-oncogene is sufficient to increase the BPTES sensitivity of MDA-MB-468 cells. Although vector-control cells showed some response to BPTES treatment, overexpression of JUN greatly sensitized cells to BPTES treatment ( Fig. 6g ). Supplementation of the medium with 1 mM dimethyl α-KG completely rescued cells from ≤12 μM BPTES, and partially rescued cells from higher BPTES concentrations ( Fig. 6g ). Although the parental and vector-control MDA-MB-468 cell lines showed little dependence on the GLS reaction, both are moderately glutamine-dependent ( Supplementary Figs 3 and 11 ). This reflects the importance of an exogenous glutamine supply for other metabolic processes that do not involve the GLS reaction, such as nucleotide biosynthesis and protein synthesis. Glutamine dependence of the JUN -overexpressing derivative cell line was unchanged from that of the parental cells ( Supplementary Fig. 11 ). c-Jun regulated transcript levels in invasive breast cancer To establish further the relationship between c-Jun activity and GLS expression in breast cancer, we used the cBioportal [45] , [46] suite of tools ( www.cbioportal.org ) to analyse data from The Cancer Genome Atlas (TCGA) Breast Invasive Carcinoma (TCGA, provisional) data set (959 samples). In many cancers, upregulation of c-Jun occurs at the post-transcriptional and post-translational levels, but not at the transcriptional level (see Discussion). Consequently, JUN mRNA levels are rarely upregulated, even though c-Jun protein levels can be highly elevated. Consistent with these findings, TCGA data showed that JUN mRNA was elevated ( z score >2.0) in only 3% of invasive breast carcinoma samples. We therefore determined whether the expression levels of some validated c-Jun transcriptional targets correlate with those of GLS . We selected only confirmed direct targets of c-Jun (and not v-Jun) that contain a c-Jun binding site within the promoter region [35] , [47] , [48] , [49] , and we eliminated from the list those c-Jun target genes that are frequently altered at the genomic level within the data set (for example, CCND1 , amplified in 16% of samples, and TP53 , mutated in 31% of samples). Using the resulting list of c-Jun targets ( Supplementary Table 2 ), we found that transcripts that are upregulated by c-Jun almost invariably correlate positively with GLS mRNA levels, whereas those targets that are transcriptionally repressed by c-Jun exhibit a negative correlation with the GLS transcript ( Fig. 7 ; see also Supplementary Figs 12 and 13 ). 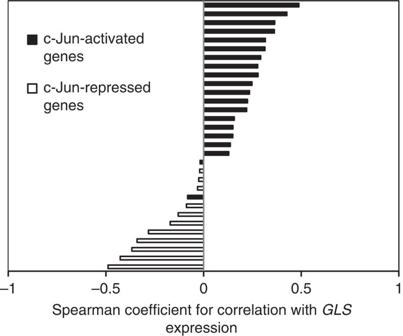Figure 7: TheGLStranscript correlates with established c-Jun target transcripts in invasive breast cancer. Bar chart showing the Spearman correlation coefficients between mRNA levels ofGLSand of established c-Jun transcriptional targets. Transcripts that are upregulated by c-Jun are shown in black, and almost exclusively correlate positively withGLS. Transcripts that are repressed by c-Jun are shown in white, and all correlate negatively withGLS. Correlation plots were prepared and correlation coefficients determined using the cBioportal suite of tools and data from The Cancer Genome Atlas (TCGA) Breast Invasive Carcinoma (TCGA, provisional) data set. Figure 7: The GLS transcript correlates with established c-Jun target transcripts in invasive breast cancer. Bar chart showing the Spearman correlation coefficients between mRNA levels of GLS and of established c-Jun transcriptional targets. Transcripts that are upregulated by c-Jun are shown in black, and almost exclusively correlate positively with GLS . Transcripts that are repressed by c-Jun are shown in white, and all correlate negatively with GLS . Correlation plots were prepared and correlation coefficients determined using the cBioportal suite of tools and data from The Cancer Genome Atlas (TCGA) Breast Invasive Carcinoma (TCGA, provisional) data set. Full size image In proliferating cells, the TCA cycle serves as a major source of biosynthetic precursors. Metabolic intermediates that are lost to anabolic pathways must be rapidly replenished, and the most abundant carbon sources for these anaplerotic reactions are glucose and glutamine. Indeed, anaplerosis is a key function underlying the upregulated consumption of these nutrients by cancer cells [10] , [11] , [50] . An important route for the delivery of glutamine-derived carbon into the TCA cycle begins with the hydrolysis of glutamine to glutamate, a reaction catalysed by glutaminase. The TCA cycle intermediate α-ketoglutarate can then be generated through the action of glutamate dehydrogenase, or through transaminase activities. In this study, we used an inducible MEF system for hyper-activating Rho GTPase signalling, which we previously linked to increased mitochondrial GLS activity in NIH-3T3 cells [20] , and also to upregulated glutamine-mediated anaplerosis for oxidative TCA cycle flux in MEFs [51] . Ectopic expression of oncogenic-Dbl in NIH-3T3 cells leads to elevated levels of the GLS transcript ( Supplementary Fig. 14a ), but the lower background level of GLS in MEFs relative to NIH-3T3 cells ( Supplementary Fig. 14b ) allows for a much clearer read-out, by RT–PCR and especially by western blot, of changes in GLS expression. By selectively inhibiting signalling pathways activated downstream of the Rho GTPases in the inducible system, we have now discovered that the c-Jun N-terminal kinase (JNK) and the oncogenic transcription factor c-Jun are critical for upregulating GLS at the transcript and protein levels. We also found that in human breast cancer cell lines, c-Jun levels correlate strongly with GLS levels and with sensitivity to the GLS inhibitor BPTES. Moreover, we determined that c-Jun directly binds the promoter of the GLS gene and increases its expression. Importantly, this not only leads to elevated mitochondrial glutaminase activity, but also causes cancer cells to become more dependent on glutamine-mediated anaplerosis. The c-Jun transcription factor is the cellular homologue of v-Jun, the transforming oncoprotein of avian sarcoma virus 17 (refs 52 , 53 ). A key role for c-Jun in both healthy and neoplastic tissue is to drive cell cycle progression, and fibroblasts derived from JUN -null mouse embryos exhibit a severe defect in proliferation [54] . The c-Jun protein is phosphorylated at the M/G1 transition [55] , and loss of c-Jun or expression of mutants defective for JNK-catalysed phosphorylation leads to a G2/M cell cycle block [56] . One transcriptional target of c-Jun is the CCND1 gene, which encodes the G1 to S phase regulator cyclin D1 (ref. 57 ). c-Jun also binds to a variant AP-1 site in the TP53 gene promoter, leading to suppression of p53 and of the p53-regulated cyclin-dependent kinase inhibitor p21 (ref. 54 ). The net effect is that c-Jun increases the activity of G1 cyclin-dependent kinase complexes. When taken together, these findings provide a biological rationale for the positive regulation of GLS by c-Jun that we describe. In order for sustained proliferation to occur, signalling to the cell cycle machinery must be coordinated with reprogramming of cellular metabolism to support biomass accumulation. By simultaneously driving cell cycle progression and upregulating GLS expression, c-Jun promotes cell proliferation and also activates TCA cycle anaplerosis to replenish metabolites that have been directed to biosynthetic pathways ( Fig. 8 ). Notably, two other reported regulators of GLS expression are involved in cell cycle control. The Rb protein prevents G1 to S phase progression [58] , and loss of this tumour suppressor leads to upregulation of GLS [41] . Similarly, the oncogenic transcription factor c-Myc promotes G1 to S phase transition, and is a positive regulator of GLS expression [22] , [23] . 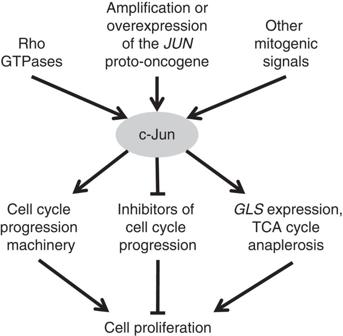Figure 8: c-Jun coordinates cell cycle progression with metabolic reprogramming. Diagram summarizes the coordinated regulation of cell proliferation by c-Jun. Transcriptional activity of c-Jun can be enhanced by activating phosphorylations downstream of mitogenic signalling pathways, including those mediated by the Rho family of GTPases. c-Jun can also be upregulated by amplification or increased expression of theJUNproto-oncogene. A key role for c-Jun is to drive cell cycle progression, which is achieved through transcriptional repression of cell cycle inhibitors and transcriptional activation of cell cycle progression machinery. In this study, we report that c-Jun also controls metabolic reprogramming to support proliferation, by upregulatingGLSexpression and thereby stimulating delivery of glutamine-derived carbon into the TCA cycle. Figure 8: c-Jun coordinates cell cycle progression with metabolic reprogramming. Diagram summarizes the coordinated regulation of cell proliferation by c-Jun. Transcriptional activity of c-Jun can be enhanced by activating phosphorylations downstream of mitogenic signalling pathways, including those mediated by the Rho family of GTPases. c-Jun can also be upregulated by amplification or increased expression of the JUN proto-oncogene. A key role for c-Jun is to drive cell cycle progression, which is achieved through transcriptional repression of cell cycle inhibitors and transcriptional activation of cell cycle progression machinery. In this study, we report that c-Jun also controls metabolic reprogramming to support proliferation, by upregulating GLS expression and thereby stimulating delivery of glutamine-derived carbon into the TCA cycle. Full size image Mirroring the ability of v-Jun to cause avian sarcoma, the JUN gene is highly amplified and overexpressed in aggressive human sarcomas [59] , and in an analysis of copy number alterations across 3,131 diverse cancer samples, JUN was found to be significantly amplified across the entire data set [60] . In many cancers, protein levels of c-Jun are highly upregulated even in the absence of JUN amplifications or elevated transcription of the JUN gene. This can be due to both translational activation and increased protein stability. For example, c-Jun is highly elevated in melanoma cells as a result of increased translation following loss of mi-R125b, which binds to the coding region of the JUN transcript and suppresses translation in normal melanocytes [61] . In breast cancer cells, c-Jun is also upregulated at the protein level but not at the transcriptional level [37] . One mechanism for this involves downregulation of the tumour suppressor COP1 E3 ubiquitin ligase, which targets c-Jun for degradation [37] . Indeed, among the cell lines used in the present study, BT-549, Hs 578T and MDA-MB-231 are reported to have low COP1 levels, whereas MCF7 and T47D have elevated COP1 (ref. 37 ). For transcriptional activity, c-Jun and related transcription factors must form a dimeric complex, which is known as AP-1 and consists of Jun–Jun or Jun–Fos dimers. Jun-family members (c-Jun, JunB and JunD) can dimerize with themselves or with Fos proteins, whereas Fos-family members (c-Fos, Fra-1, Fra-2 and FosB) must heterodimerize with a Jun protein [57] . This raises some questions concerning the fine-tuning of GLS regulation. Of the AP-1 transcription factors, c-Jun is the most potent transcriptional activator. However, Jun-Fos heterodimers are more stable and efficient at driving transcriptional activation than Jun–Jun dimers [57] . Importantly, the promoter specificity of dimers containing c-Jun differs according to the dimerization partner, and the relative abundances of potential partners vary between cell types [62] , [63] . Consequently, the Jun- and Fos-family members that are expressed within a given cell likely influence the regulation of GLS expression by c-Jun, and it is possible that JunB or JunD might substitute for c-Jun in some contexts. High levels of c-Jun are associated with aggressive, invasive and metastatic behaviour in breast cancer. Ectopic overexpression of JUN in the MCF7 cell line leads to increased invasion and tumorigenicity, whereas a dominant-negative variant of c-Jun causes cell cycle arrest [64] , [65] . Several studies have found that c-Jun is specifically elevated in triple-negative breast cancer (TNBC) cells [35] , [37] , [66] and MYC expression is also reported to be upregulated in TNBC [67] . This could explain why TNBC cell lines have higher GLS levels and greater sensitivity to the GLS inhibitor CB-839 (a BPTES derivative) than receptor-positive breast cancer cells [21] . In conclusion, we have identified a JNK/c-Jun-dependent signalling pathway that is responsible for upregulating GLS levels during cellular transformation. Moreover, we show that the c-Jun transcription factor is an important regulator of GLS expression in breast cancer, and can drive cellular dependence on the glutaminase reaction, thus conferring sensitivity to the GLS inhibitor BPTES. Our findings link a key player in cell cycle progression with a metabolic pathway that supports cell proliferation, and illustrate that re-programming of cellular metabolism is intricately connected with oncogenic transformation. Furthermore, our work reveals a novel function for the c-Jun oncoprotein in cancer, and suggests why certain types of cancer such as triple-negative breast cancer might be more susceptible to glutaminase-targeted therapy. Isogenic inducible MEF system for oncogenic-Dbl expression The inducible MEF line used in this study was generated as described previously [51] . Briefly, the gene encoding oncogenic-Dbl was sub-cloned into vector pTRE-HA (Clontech). Parental MEFs containing the transcriptional transactivator tTA (Clontech) were then co-transfected with the resulting pTRE-HA-onco-Dbl vector along with vector pMET-puro, in a 20:1 ratio. Following puromycin selection ( ∼ 3 weeks), colonies were screened for inducible expression of oncogenic-Dbl. Cells were maintained at 37 °C, 5% CO 2 atmosphere, in DMEM medium containing 4 mM glutamine (Gibco) and supplemented with 10% (v/v) tetracycline-free FBS (Gibco) and 0.6 μg ml −1 doxycycline. Expression of oncogenic-Dbl was induced by re-plating cells in doxycycline-free medium (10% FBS). Residual doxycycline was removed by replacing the medium (with the appropriate concentration of FBS, and small-molecule inhibitor where relevant) after 5 h. Uninduced control samples were treated in the same way: re-plating followed by media change at 5 h, but with 0.6 μg ml −1 doxycycline present at all times. For glutamine-withdrawal experiments, glutamine-free DMEM medium (Gibco) was supplemented with dialysed FBS (Gibco). Growth medium containing other concentrations of glutamine was prepared by mixing appropriate volumes of DMEM (4 mM glutamine) and glutamine-free DMEM. Breast cancer cell culture and media Breast cancer cell lines ZR-75-1, BT-474, CAMA-1, SK-BR-3, T-47D, MCF7, MDA-MB-468, BT-549, Hs 578T, MDA-MB-453 and MDA-MB-231 were obtained from the American Type Cell Culture Collection (ATCC). The TSE breast cancer cell line was kindly supplied by Dr Steven Abcouwer (University of Michigan). All breast cancer cell lines were maintained at 37 °C, 5% CO 2 atmosphere, in RPMI 1640 medium containing 2 mM glutamine (Gibco) and supplemented with 10% FBS (Gibco). For glutamine-withdrawal experiments, glutamine-free RPMI 1640 medium (Gibco) supplemented with 10% dialysed FBS (Gibco) was used. Cell lines were periodically tested for Mycoplasma contamination. DNA constructs DNA primers were synthesized by Integrated DNA Technologies. Plasmid pCDNA3.1/V5-His TOPO was purchased from Life Technologies. The JUN gene was PCR amplified from plasmid pMIEG3-c-Jun, which was a gift from Alexander Dent (Addgene plasmid # 40348) [68] , using primers JUN_AMP_F (5′-TTATGGATCCATGACTGCAAAGATGGAAACGACC-3′) and JUN_AMP_R (5′-TTATGATATCAAATGTTTGCAACTGCTGCGTTAGC-3′), which added a BamH1 site and EcoRV site, respectively. The PCR product was purified (QIAquick PCR purification kit, QIAGEN), digested with BamH1 and EcoRV (New England Biolabs), re-purified and ligated (T4 DNA ligase, New England Biolabs) into pre-digested and purified pCDNA3.1/V5-His TOPO to yield an expression vector for JUN-V5 , pCDNA3.1-JUN. The construct was verified by sequencing. The plasmids pCDNA3 Flag MKK7B2Jnk1a1 (Addgene plasmid # 19726) [34] , pCDNA3 Flag MKK7B2Jnk2a2 (Addgene plasmid # 19727) [34] and pCDNA3 Flag MKK7B2Jnk3a2 (Addgene plasmid # 19729) [34] were all gifts from Roger Davis. Antibodies and reagents Antibodies recognizing the following proteins were purchased from Cell Signaling Technology: HA-tag (cat. no. 3724) used at 1:5,000, α/β-tubulin (cat. no. 2148) used at 1:5,000, phospho-SEK1/MKK4 (S257) (cat. no. 4514) used at 1:2,000, phospho-MKK7 (S271/T275) (cat. no. 4171) used at 1:2,000, phospho-JNK (T183/Y185) (cat. no. 4668) used at 1:2,000, phospho-c-Jun (S73) (cat. no. 3270) used at 1:2,000, c-Jun (cat. no. 9165) used at 1:2,000, JunB (cat. no. 3753) used at 1:2,000, JunD (cat. no. 5000) used at 1:2,000, phospho-p38 MAPK (T180/Y182) (cat. no. 4511) used at 1:2,000, p38 MAPK (cat. no. 8690) used at 1:2,000, phospho-ERK1/2 (T202/Y204) (cat. no. 4370) used at 1:2,000, ERK1/2 (cat. no. 9102) used at 1:2,000, phospho-myosin light chain 2 (S19) (cat. no. 3675) used at 1:1,000, myosin light chain 2 (cat. no. 3672) used at 1:1,000, phospho-AMPKα (T172) (cat. no. 4188) used at 1:2,000, AMPKα (cat. no. 2603) used at 1:2,000, phospho-Akt (T308) (cat. no. 9275) used at 1:2,000, Akt (cat. no. 9272) used at 1:2,000, phospho-p70 S6 kinase (T389) (cat. no. 9205) used at 1:2,000, p70 S6 kinase (cat. no. 9202) used at 1:2,000, STAT1 (cat. no. 9172) used at 1:2,000, Rb (cat. no. 9309) used at 1:2,000, Glut1 (cat. no. 12939) used at 1:4,000, and c-Myc (cat. no. 5605) used at 1:2,000. The antibody recognizing GLS was purchased from Abgent (cat. no. AP8809b) and used at 1:8,000. Clarification of the bands recognized by this antibody is shown in Supplementary Fig. 15 . Antibodies recognizing MKK4 (MEK4) (cat. no. ab33912), MKK7 (MEK7) (cat. no. ab52618) and phospho-c-Myc (T58+S62) (cat. no. ab10568), all used at 1:4,000, were purchased from Abcam. Antibodies recognizing JNK (cat. no. sc-571) and GLUD1/2 (cat. no. sc-160383), both used at 1:2,000, were purchased from Santa Cruz Biotechnology. The antibody recognizing V5-tag was purchased from Life Technologies (cat. no. R960) and used at 1:5,000. Secondary antibodies used, as appropriate, were Cell Signaling Technology anti-rabbit IgG, HRP-linked (cat. no. 7074) or anti-mouse IgG, HRP-linked (cat. no. 7076), or Santa Cruz Biotechnology donkey anti-goat IgG-HRP (cat. no. sc-2020). BPTES was synthesized and kindly provided by Dr Scott Ulrich, Ithaca College. ROCK inhibitor Y-27632 (10 mM solution in DMSO), the JNK inhibitor SP600125 (50 mM solution in DMSO) and G418 were purchased from Calbiochem. All other reagents were purchased from Sigma-Aldrich unless otherwise stated. Western blot analysis Whole-cell lysates were prepared in lysis buffer (50 mM HEPES pH 8.0, 150 mM NaCl, 1 mM Na 3 VO 4 , 25 mM NaF, 1% (v/v) Triton X-100, 1 mM MgCl 2 , 50 mM β-glycerophosphate, 30 μg ml −1 leupeptin, 5 μg ml −1 aprotinin) and insoluble debris was pelleted by centrifugation and removed. Protein concentration was determined by Bradford assay (Bio-Rad), and lysate proteins denatured by boiling for 5 min in reducing SDS-sample buffer. Lysate proteins (20 μg total protein/lane) were then resolved on Novex 4–20% Tris-glycine mini or midi protein gels (Life Technologies), and transferred to polyvinylidene difluoride membranes (PerkinElmer). Membranes were blocked in 7% bovine serum albumin in tris-buffered saline and tween 20 (TBST) for 1 h at room temperature, and probed overnight at 4 °C in primary antibody solution (manufacturer recommended concentration) in TBST. They were then washed in TBST, and incubated in TBST solution containing 25% (v/v) non-fat dry milk powder and appropriate secondary antibody at the manufacturer’s recommended concentration for 1 h. Finally, the membranes were washed in TBST, and bands imaged using Western Lightning Plus-ECL (PerkinElmer) and HyBlot ES autoradiography film (Denville Scientific Inc.). MEF saturation density analysis DMEM medium supplemented with 10% FBS±0.6 μg ml −1 doxycycline was added to 60 mm dishes (3 ml per dish), and dishes were then seeded with 1 × 10 5 MEFs per dish. Following cell attachment (5 h), growth medium was replaced with fresh medium containing appropriate supplements. Growth medium was subsequently replaced at 48 h intervals. At day 8, growth medium was removed and 1.5 ml 3.7% formaldehyde solution in H 2 O was added for 30 min. The formaldehyde solution was removed, and 1.5 ml crystal violet solution was added for 20 min at room temperature. This was then removed, and dishes washed four times with 3 ml H 2 O and allowed to dry before imaging. MEF anchorage-independent growth assay Uninduced or oncogenic-Dbl-induced MEFs were seeded at a density of 8,000 cells per ml in medium containing 0.3% (w/v) agarose, onto underlays of medium containing 0.6% agarose, in six-well plates. Both layers of medium were supplemented with appropriate concentrations of doxycycline (uninduced cells) and BPTES. Cultures were fed every 3 days, and the total number of colonies was counted after 15 days. Cell proliferation assays Culture medium supplemented with glutamine or with inhibitors at the described concentrations was added to 12-well plates (1 ml per well), and wells were seeded with cells at day 0 as follows (numbers optimized to avoid over-confluence during the assay). TSE cells: 5 × 10 3 cells per well. MDA-MB-231, MDA-MB-453, MDA-MB-468, BT-549: 1 × 10 4 cells per well. Hs 578T, MCF7, T-47D, CAMA-1, SK-BR-3, BT-474: 1.5 × 10 4 cells per well. ZR-75-1: 2 × 10 4 cells per well. Following cell attachment, growth medium was replaced at 12 h and subsequently every 48 h. At day 6, cells were trypsinized, suspended in an appropriate volume of medium, and a hemacytometer was used to determine the total number of cells per well. All cell proliferation assays were carried out in triplicate, and the mean and s.d. calculated. Mitochondrial isolation Mitochondria were isolated using the Qproteome mitochondria isolation kit (QIAGEN), following the manufacturer’s instructions. For MEFs grown in low-serum media, 3 × 15 cm dishes of cells at ∼ 70% confluency were collected, and for MDA-MB-468 cells, 2 × 15 cm dishes of cells at ∼ 70% confluency were collected. The total protein of the starting material (collected cells) and of the isolated mitochondria suspension was measured by Bradford assay (Bio-Rad). This allowed glutaminase activity to be determined per unit of total cellular protein (see below). Mitochondrial glutaminase activity assay A two-step protocol was used to assay glutaminase activity, as previously described [28] . In the first reaction, glutaminase catalyses the hydrolysis of glutamine to glutamate, and in the second reaction glutamate dehydrogenase catalyses the oxidative deamination of glutamate to form α-ketoglutarate and NADH, which can be measured through its absorbance at 340 nm. Briefly, mitochondria (10 μg total protein) were added to 105 μl of reaction mix 1 (20 mM glutamine, 0.2 mM EDTA, 50 mM Tris-acetate, pH 8.6). Samples were rotated at 37 °C for 45 min. The reaction was then quenched by adding 10 μl of 3 M HCl, and samples were placed on ice. Next, 20 μl of reaction mix 1 was added to 200 μl of reaction mix 2 (1 unit bovine liver glutamate dehydrogenase (Sigma-Aldrich), 80 mM Tris-HCl pH 9.4, 200 mM hydrazine, 0.25 mM ADP, 2 mM NAD). The samples were mixed and incubated for 1 h at room temperature. The A 340 was then determined against a blank in which a heat-inactivated mitochondrial sample was added to reaction mix 1. A standard curve was also prepared by adding known amounts of glutamate to reaction 2. This allowed the amount of glutamate generated during reaction 1 to be determined. All assays were carried out in triplicate, and the mean and s.d. calculated. Real-time PCR analysis Total RNA was extracted from cells using the RNeasy mini kit (QIAGEN), and cDNAs were prepared using the SuperScript III first-strand synthesis system (Life Technologies). RT-PCR was carried out using the 7,500 fast real-time PCR system (Applied Biosystems), with cDNA as a template and GLS primers GLS-F (5′-TGTCACGATCTTGTTTCTCTGTG-3′) and GLS-R (5′-TCATAGTCCAATGGTCCAAAG-3′). Primers for mouse GAPDH (mGAPDH-F, 5′-ACAGTCCATGCCATCACTGCC-3′ and mGAPDH-R, 5′-GCCTGCTTCACCACCTTCTTG-3′) or human ACTB (hACTB-F, 5′-CATCGAGCACGGCATCGTCA-3′ and hACTB-R, 5′-TAGCACAGCCTGGATAGCAAC-3′) were used as endogenous controls, as appropriate. All reactions were carried out using POWER SYBR green PCR master mix (Life Technologies). At least three replicates of each PCR were carried out. Chromatin immunoprecipitation Chromatin immunoprecipitations were performed using the SimpleChIP enzymatic chromatin IP kit (Cell Signaling Technology), following the manufacturer’s instructions. MDA-MB-231 cells (5 × 15 cm dishes at ∼ 85% confluency) were used as the source of chromatin. Analysis following chromatin digestion showed that DNA was digested to fragments of the desired size (150–900 bp, equivalent to 1–5 nucleosomes). An antibody against endogenous c-Jun (Cell Signaling Technology, 9165) was used to immunoprecipitate complexes containing c-Jun. Following reversal of protein–DNA complexes and purification of DNA, RT–PCR was carried out as described above but using the purified DNA as a template. Three primer sets were designed to amplify 100–200 bp fragments centred on the putative c-Jun binding site of the GLS promoter at position −188 bp relative to the TSS. Set 1 (forward and reverse): 5′-CCCTAGTACCCAACTAGGCTAGCC-3′ and 5′-CCTCTCTTTTGATTGGCGATTAGGG-3′. Set 2 (forward and reverse): 5′-GCGTGCAGAAAGTGGCTACTGAGC-3′ and 5′-CTCTCGGCTCTGGGTGCGCGGAGAG-3′. Set 3 (forward and reverse): 5′-CCTCGGAGTTGGCACGGCGTGCAG-3′ and 5′-GGCAGTCAAATTTCTCTCGGCTC-3′. RNA interference Knockdown of JUN expression in BT-549 cells was achieved using Silencer select pre-designed and validated siRNA (Life Technologies). Because endogenous c-Jun levels are so high in this cell line, two rounds of siRNA treatment were required to achieve effective knockdowns. Two siRNA products (manufacturer ID # s7658 and s7659) were used, along with the Silencer select negative control no. 1 siRNA. Transfections were carried out in 10 cm dishes at ∼ 80% confluency using Lipofectamine 2000 transfection reagent (Life Technologies) and following the manufacturer’s instructions. The final siRNA concentration was 15 nM in all cases. Transfection medium was replaced with fresh growth medium 5 h after treatment. At 48 h following the initial transfection, the procedure was repeated, and cells were collected after a further 48 h. Stable cell lines Transfection of breast cancer cell lines with plasmid DNA constructs (pCDNA3.1 or pCDNA3.1-JUN) was carried out using Lipofectamine 2000 transfection reagent (Life Technologies), following the manufacturer’s instructions. At 48 h after transfection, cells were placed under G418 selection by supplementing the growth medium with G418 (500 μg ml −1 for MCF7, and 800 μg ml −1 for MDA-MB-468). Growth medium was replaced every 48 h for 2–3 weeks, until isolated colonies ( ∼ 2 mm diameter) were apparent on the plate. At this point, individual clones were transferred to 12-well dishes and expanded in 250 μg ml −1 G418 for further analysis. Appropriate clones were screened for c-Jun-V5 by western blot, and V5-positive clones were maintained in 250 μg ml −1 G418. TCGA data The Cancer Genome Atlas (TCGA) Breast Invasive Carcinoma (TCGA, provisional) data set was accessed, all data were analysed, and correlation plots prepared using the cBioportal [45] , [46] suite of tools ( www.cbioportal.org ). Statistical analyses All differences were analysed with Student’s t -test. A P value <0.05 was considered to be significant and marked (*), and a P value below 0.01 was considered to be highly significant and marked (**). How to cite this article: Lukey, M. J. et al. The oncogenic transcription factor c-Jun regulates glutaminase expression and sensitizes cells to glutaminase-targeted therapy. Nat. Commun. 7:11321 doi: 10.1038/ncomms11321 (2016).